Modulation of rod photoreceptor output by HCN1 channels is essential for regular mesopic cone vision Retinal photoreceptors permit visual perception over a wide range of lighting conditions. Rods work best in dim, and cones in bright environments, with considerable functional overlap at intermediate (mesopic) light levels. At many sites in the outer and inner retina where rod and cone signals interact, gap junctions, particularly those containing Connexin36, have been identified. However, little is known about the dynamic processes associated with the convergence of rod and cone system signals into ON- and OFF-pathways. Here we show that proper cone vision under mesopic conditions requires rapid adaptational feedback modulation of rod output via hyperpolarization-activated and cyclic nucleotide-gated channels 1. When these channels are absent, sustained rod responses following bright light exposure saturate the retinal network, resulting in a loss of downstream cone signalling. By specific genetic and pharmacological ablation of key signal processing components, regular cone signalling can be restored, thereby identifying the sites involved in functional rod–cone interactions. In retinal photoreception, the highly light-sensitive rods respond to weak stimuli under dim light conditions (scotopic vision) but saturate under bright light conditions, whereas the less sensitive cones require stronger stimuli but continue to function under bright light (photopic) conditions. Both photoreceptor types contribute to vision under intermediate (mesopic) conditions [1] , [2] . Anatomically, the major rod and cone pathways in the retina are well established ( Fig. 1 ). Cones connect to ON- and OFF-cone bipolar cells, which in turn connect to ON- and OFF-ganglion cells. Rod signals feed into both ON- and OFF-channels in the inner retina via rod bipolar and AII-amacrine cells (primary rod pathway), or via cone bipolar cells that the rods access through gap junctional connections between rods and cones in the outer retina (secondary rod pathway) that contain connexin 36 (refs 3 , 4 , 5 , 6 , 7 , 8 ). A third pathway connecting rods to certain types of OFF bipolar cells [9] , [10] , [11] , [12] awaits further clarification and was, therefore, not included in the schematic diagram. 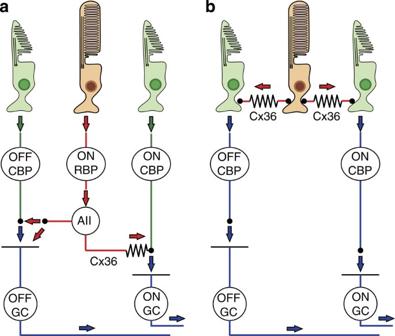Figure 1: Schematic diagram of rod and cone pathways in the mammalian retina. Rod and cone signals converge at different sites in the retina. (a) In the classical (primary) rod pathway, rod signals are conveyed via the rod bipolar cell (ON-RBP) onto the AII-amacrine cell. The AII provides electrical input via Cx36 containing gap junctions into ON-cone bipolar cells (ON-CBP) and via glycinergic synapses into the OFF-pathway (OFF-cone bipolar cells, OFF-CBP and OFF-GC). (b) In the secondary rod pathway, rods feed directly into cones via Cx36 containing gap junctions. A tertiary pathway, of unknown significance, has been described that enables rods to make direct contacts to certain OFF-CBPs via chemical synapses. This pathway was omitted here for the sake of clarity. Red or green figure elements indicate signals of exclusive rod or cone origin, respectively. Blue figure elements indicate signals potentially reflecting both rod and cone activity. Figure 1: Schematic diagram of rod and cone pathways in the mammalian retina. Rod and cone signals converge at different sites in the retina. ( a ) In the classical (primary) rod pathway, rod signals are conveyed via the rod bipolar cell (ON-RBP) onto the AII-amacrine cell. The AII provides electrical input via Cx36 containing gap junctions into ON-cone bipolar cells (ON-CBP) and via glycinergic synapses into the OFF-pathway (OFF-cone bipolar cells, OFF-CBP and OFF-GC). ( b ) In the secondary rod pathway, rods feed directly into cones via Cx36 containing gap junctions. A tertiary pathway, of unknown significance, has been described that enables rods to make direct contacts to certain OFF-CBPs via chemical synapses. This pathway was omitted here for the sake of clarity. Red or green figure elements indicate signals of exclusive rod or cone origin, respectively. Blue figure elements indicate signals potentially reflecting both rod and cone activity. Full size image Although the connections between rod and cone pathways have been verified using anatomical and electrophysiological approaches in vitro , the functional consequences for vision are not entirely clear. In particular, there is a lack of understanding about how rod and cone photoreceptor signals interact in the retina when both systems are active simultaneously. Mesopic conditions, where rod and cone signals converge onto the same downstream cells, allow us to investigate how they may influence and/or modulate each other. To explore such interactions, mouse mutants deficient in hyperpolarization-activated and cyclic nucleotide-gated channels 1 (HCN1 (ref. 13 )) can be used. In photoreceptors ( Fig. 2a ), stimulation by light diminishes the dark current in the outer segments ( Fig. 2b ) by closure of cyclic nucleotide-gated channels, thereby causing a hyperpolarization of the membrane. This leads to a strongly reduced synaptic activity and a large electroretinogram (ERG) signal during the early phase shortly after a flash ( Fig. 2c ). The change in membrane potential is sensed by the HCN1 channels, but there is a certain time delay before they become active, and thus the ERG signal is initially not different between wild-type (WT) and HCN1-deficient animals. After this short delay, the associated voltage change leads to an increase in the fraction of open HCN1 channels located in the membrane of photoreceptor inner segments, causing an inward current that drives the membrane potential back towards the resting state ( Fig. 2d ). The result is a substantial, but not complete, reduction of rod output (that is, an increase in synaptic activity) in a voltage-dependent manner, apparently precluding a saturation of the downstream retinal network. 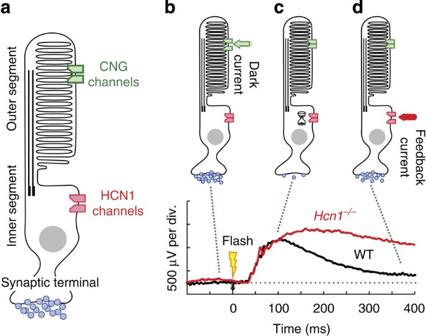Figure 2: Role of HCN1 channels in rod photoreceptor signal generation. Location and functional role of HCN1 channels in rod photoreceptors. Corresponding Ganzfeld ERG traces are shown to point out the functional impact of the state changes of HCN1 and CNG channels. (a) Sketch of a rod photoreceptor. Cyclic-nucleotide gated (CNG) and HCN1 channels are highlighted, together with the state of synaptic activity indicated by the amount of transmitter vesicle release. (b) Dark state. CNG channels in the outer segment are open and HCN1 channels in the inner segment are closed. The resulting synaptic activity is high, which translates into a baseline ERG signal. (c) Early phase shortly after a flash. CNG channels close, leading to an initially strongly reduced synaptic activity and to a large ERG signal. HCN1 channels show a certain time delay and are not yet active, signified by the hour glass symbol. (d) Later phase after a flash. HCN1 channels open and their feedback current diminishes the membrane voltage, leading to an increase in synaptic activity despite unchanged CNG channel status. The ERG amplitude is reduced in WT animals, but not in HCN1 channel-deficient animals lacking this feedback mechanism. Figure 2: Role of HCN1 channels in rod photoreceptor signal generation. Location and functional role of HCN1 channels in rod photoreceptors. Corresponding Ganzfeld ERG traces are shown to point out the functional impact of the state changes of HCN1 and CNG channels. ( a ) Sketch of a rod photoreceptor. Cyclic-nucleotide gated (CNG) and HCN1 channels are highlighted, together with the state of synaptic activity indicated by the amount of transmitter vesicle release. ( b ) Dark state. CNG channels in the outer segment are open and HCN1 channels in the inner segment are closed. The resulting synaptic activity is high, which translates into a baseline ERG signal. ( c ) Early phase shortly after a flash. CNG channels close, leading to an initially strongly reduced synaptic activity and to a large ERG signal. HCN1 channels show a certain time delay and are not yet active, signified by the hour glass symbol. ( d ) Later phase after a flash. HCN1 channels open and their feedback current diminishes the membrane voltage, leading to an increase in synaptic activity despite unchanged CNG channel status. The ERG amplitude is reduced in WT animals, but not in HCN1 channel-deficient animals lacking this feedback mechanism. Full size image In this study, by examining transgenic mice devoid of HCN1 channels that were exposed to bright stimuli under mesopic conditions, we found that the lack of modulation of rod output lead to large, prolonged signals that saturated the retinal circuits, thereby obscuring postreceptoral cone system responses. This was verified both in the ERG reflecting transient retinal signals in vivo , and in patch–clamp recordings of retinal ganglion cells (GCs) in vitro , whose output goes to higher brain regions. Using a combined approach of specific double knockout mutants and pharmacological blockade, we were able to identify the sites of normal interaction between rod and cone signals in both outer and inner retina. Our study shows that HCN1 channels are essential for vision under mesopic conditions and reveals the mechanisms by which the pathologically increased and prolonged rod responses in HCN1 −/− mice lead to a disturbance of physiologically normal rod–cone interactions. HCN1 −/− mice do not resolve high-frequency mesopic stimuli In ERG recordings, we maintained mesopic conditions (where both rod and cone systems were active in processing light input simultaneously) by trains of bright flashes (2 cd · s m −2 ; Fig. 3a,b ). On the basis of a previous work [14] (and our unpublished data with this protocol in nob mice, N.T. and M.W.S), we knew that responses to low temporal frequency stimulation (0–3 Hz) are dominated by rod system activity, those to intermediate frequency stimulation (3–15 Hz) by cone ON system activity, and those to high-frequency stimulation (≥15 Hz) by cone OFF system activity [15] , [16] . 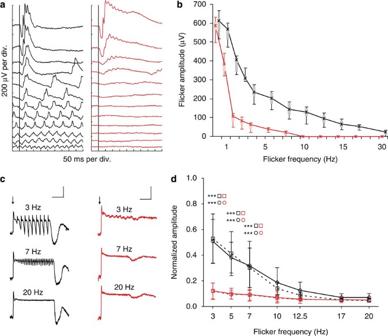Figure 3: Profound alterations of the flicker frequency response in HCN1−/−mice. (a) Comparison of flicker ERGs of WT (black) and HCN1−/−(red) mice at a flash intensity of 0.5 log cd s m−2. In the mutants, the rod-dominated low frequency part shows prolonged response waveforms, and, strikingly, any cone-related signals are missing over the entire frequency range. Flicker frequencies from top to bottom were 0.5, 1, 2, 3, 5, 7, 10, 12, 15, 18, 20 and 30 Hz. (b) Box-and-whisker plot of flicker ERG response amplitudes as in (a) in WT (black,n=4) and HCN1−/−(red,n=4) mice. Boxes indicate the 25 and 75% quantile range; whiskers indicate the 5 and 95% quantiles; and the asterisks indicate the median of the data. (c) OFF-GC current responses to mesopic flicker stimuli in the WT and HCN1−/−retina. The onset of stimulation is indicated by an arrow. Flash duration: 20 ms. Flash intensity: 760 rhodopsin isomerizations per rod and flash (Rh* per rod*flash). Stimulus duration: 3 s (3 Hz), 3.5 s (7 and 20 Hz). Scale bars: horizontal 1s; vertical WT 0.5 nA, HCN1−/−0.2 nA. (d) Resolution of flicker stimuli of GCs in the WT (black) and HCN1−/−(red) retina. ON-GCs (circles, solid lines) and OFF-GCs (squares, broken lines) were analysed separately (black circles,n=8; red circles,n=9; black squares,n=23; red squares,n=25). The normalized response amplitude (average current amplitudes evoked in response to single flashes were normalized to the maximum current amplitude of the response) is plotted against the stimulation frequency (note that GC data start at 3 Hz, whereas ERG data (a,b) start at 0.5 Hz). Error bars indicate±s.d. around the mean. As in thein vivoelectrophysiology (a,b), normalized response amplitudes of both ON- and OFF-GCs differed considerably between WT and HCN1−/−retina; these differences reached statistical significance up to a stimulation frequency of 7 Hz (P<0.001; 2-way ANOVA). Figure 3: Profound alterations of the flicker frequency response in HCN1 −/− mice. ( a ) Comparison of flicker ERGs of WT (black) and HCN1 −/− (red) mice at a flash intensity of 0.5 log cd s m −2 . In the mutants, the rod-dominated low frequency part shows prolonged response waveforms, and, strikingly, any cone-related signals are missing over the entire frequency range. Flicker frequencies from top to bottom were 0.5, 1, 2, 3, 5, 7, 10, 12, 15, 18, 20 and 30 Hz. ( b ) Box-and-whisker plot of flicker ERG response amplitudes as in ( a ) in WT (black, n =4) and HCN1 −/− (red, n =4) mice. Boxes indicate the 25 and 75% quantile range; whiskers indicate the 5 and 95% quantiles; and the asterisks indicate the median of the data. ( c ) OFF-GC current responses to mesopic flicker stimuli in the WT and HCN1 −/− retina. The onset of stimulation is indicated by an arrow. Flash duration: 20 ms. Flash intensity: 760 rhodopsin isomerizations per rod and flash (Rh* per rod*flash). Stimulus duration: 3 s (3 Hz), 3.5 s (7 and 20 Hz). Scale bars: horizontal 1s; vertical WT 0.5 nA, HCN1 −/− 0.2 nA. ( d ) Resolution of flicker stimuli of GCs in the WT (black) and HCN1 −/− (red) retina. ON-GCs (circles, solid lines) and OFF-GCs (squares, broken lines) were analysed separately (black circles, n =8; red circles, n =9; black squares, n =23; red squares, n =25). The normalized response amplitude (average current amplitudes evoked in response to single flashes were normalized to the maximum current amplitude of the response) is plotted against the stimulation frequency (note that GC data start at 3 Hz, whereas ERG data ( a , b ) start at 0.5 Hz). Error bars indicate±s.d. around the mean. As in the in vivo electrophysiology ( a , b ), normalized response amplitudes of both ON- and OFF-GCs differed considerably between WT and HCN1 −/− retina; these differences reached statistical significance up to a stimulation frequency of 7 Hz ( P <0.001; 2-way ANOVA). Full size image The ERG data in Figure 3a,b show that low frequency stimuli were well resolved in HCN1 −/− mice despite considerably prolonged responses, whereas, to our surprise, response amplitudes decreased dramatically with increasing frequency, and essentially no responses were observable above 5 Hz. In this assay, there was no sign of any cone system activity in HCN1 −/− mutants, either in the ON or the OFF pathway, despite the fact that cones were found to be functional in HCN1 −/− mutants in other paradigms [13] (confirmed by our findings below). In fact, the data closely resembled those of rod-only models like CNGA3 −/− lacking the cone cyclic nucleotide-gated channel subunit A3 and, therefore, having no functional cones [15] , [16] . An important question was whether the lack of cone-driven activity observed in the ERG would also be present in the retinal output via ON- and OFF-GCs. GC responses were recorded in the whole-cell patch–clamp mode in dark-adapted whole mount preparations. Figure 3c shows representative light responses of OFF-GCs from WT and HCN1 −/− mice stimulated with mesopic flicker stimuli of 3, 7 and 20 Hz. At the onset of stimulation, the WT cell responded with a transient outward current followed by a sustained component. At 3 Hz, each subsequent flash elicited characteristic current fluctuations consisting of an initial fast and small outward current followed by a pronounced transient inward current riding on top of the sustained current. Increasing the flicker frequency to 7 Hz reduced the amplitude of the current deflection. At 20 Hz, only the sustained outward current remained. The offset of the flicker stimulus elicited a pronounced inward current (OFF-response). In the OFF-GC of the HCN1 −/− retina, the transient outward current at stimulus onset was similar to that of WT OFF-GCs; however, already at 3 Hz, light-induced current fluctuations were strongly diminished and only the sustained outward current persisted ( Fig. 3c ). Moreover, the cell did not respond with an OFF-response at the offset of the flicker stimulus. In some OFF-cells of the HCN1 −/− retina, small current deflections could be observed roughly 3 s after stimulus onset. Notably, they occurred during the flicker stimulation and did not correlate with stimulus offset. The origin of these currents is unknown. On stimulus offset, it took roughly 3 s before the outward current had completely returned to the holding level. ON-GCs of the HCN1 −/− retina had a comparably reduced ability to follow higher frequency flicker ( Fig. 3d ). In current clamp recordings, mesopic flicker stimuli induced long-lasting inhibition in OFF-GCs but long-lasting excitation in ON-GCs. In summary, a significant loss of high-frequency flicker resolution in both ON- and OFF-GCs was found in HCN1 −/− mice ( Fig. 3d ). Flicker resolution was slightly compromised for flashes of 20 rhodopsin isomerizations per rod and flash (rh* per rod flash) and was fully lost at 100–300 rh* per rod flash. These results confirm that the lack of cone signalling observed in the ERG was also characteristic of GC responses at the output level of the retina. We conclude that HCN1 channels have an important role in mesopic vision, most probably by preventing saturation of the pathways receiving input from the rod system. HCN1 −/− mice cannot follow high-intensity 6 Hz flicker A different paradigm that provides information about cone activity in the presence of rod system saturation is the 6-Hz scotopic flicker intensity series [17] , [18] . In this approach, a flicker stimulus of 6 Hz is presented with light intensity increasing in 1/5th logarithmic steps from very dim to very bright. At low and intermediate flash intensities, the recordings from WT animals ( Fig. 4a ) were dominated by the almost sinusoidal rod system responses. At high flash intensities, the more triangular cone system responses dominated. Plotting the flicker amplitude versus the stimulus intensity yields a biphasic curve in WT animals ( Fig. 4b ). A pronounced rod peak occurred around 0.01 cd s m −2 (green arrowhead) and a cone shoulder was present for the strongest stimuli (blue arrowhead). The two response regions were separated near 1 cd s m −2 by a trough that was shaped by the transition from rod to cone system dominance. 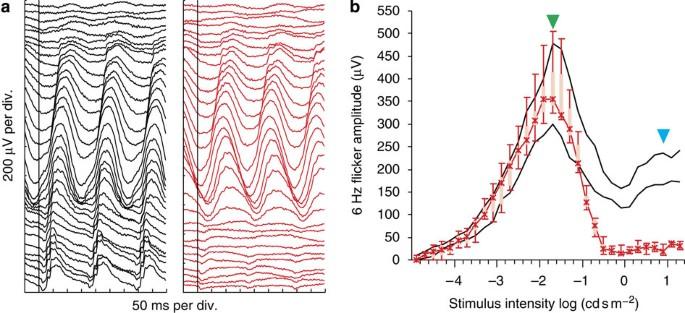Figure 4: Absence of regular cone system responses in HCN1−/−animals in the ERG 6 Hz intensity series. (a) Comparison of representative records between HCN1−/−mice (red) and WT controls (black). Traces span an intensity range of 0.000012−19 cd · s m−2from top to bottom, in steps of 0.2 logarithmic units. (b) Box-and-whisker plot of HCN1−/−mouse ERG amplitudes as in (a) in comparison to WT mouse data (each groupn=4). In the mutants, the first peak dominated by the rod system (green arrowhead) remained unchanged, whereas a considerable amplitude reduction was observed at high intensities, dominated typically by the cone system (blue arrowhead). Figure 4: Absence of regular cone system responses in HCN1 −/− animals in the ERG 6 Hz intensity series. ( a ) Comparison of representative records between HCN1 −/− mice (red) and WT controls (black). Traces span an intensity range of 0.000012−19 cd · s m −2 from top to bottom, in steps of 0.2 logarithmic units. ( b ) Box-and-whisker plot of HCN1 −/− mouse ERG amplitudes as in ( a ) in comparison to WT mouse data (each group n =4). In the mutants, the first peak dominated by the rod system (green arrowhead) remained unchanged, whereas a considerable amplitude reduction was observed at high intensities, dominated typically by the cone system (blue arrowhead). Full size image In HCN1 −/− mice, rod system responses at low and intermediate flash intensities were broader than those of WT animals ( Fig. 4a ), but had normal amplitudes ( Fig. 4b ; well between the 5 and 95% quartiles of WT). However, at the higher intensities usually dominated by cone system responses, deflections vanished almost entirely, corroborating the previous observation of a cone system deficiency ( Fig. 3 ). The only cone system activity observed for the high-intensity stimulation was some tiny negative spikes in the traces, which we interpreted to be potential cone a-waves (that is, signs of photoreceptor activity without activation of the respective bipolar cells). The presumed cone a-waves in the 6-Hz flicker data provided further support that cones in HCN1 −/− mice were functional. However, in the mesopic range, when both rod and cone photoreceptors were active, no signals originating from the cone system were observed at the level of the bipolar cells (assessed by ERG) or ganglion cells. Rod system saturation suppresses cone system signalling Rod and cone signals converge at several sites in the retina ( Fig. 1a,b ). Large rod responses, that occur at higher mesopic levels, might, at each site, saturate the respective part of the pathway and, thereby, prevent cone signals from being passed on to subsequent neurons. This may be facilitated by the fact that, under such experimental conditions, cone system responses are commonly slower than rod system responses. The cone signals therefore can not excite downstream neurons that are already active because of previous stimulation originating from the rod system. We suggest that in WT animals, the internal feedback mediated by HCN1 channels in rod photoreceptors prevents such pathway saturation by modulating rod synaptic output. In contrast, in the absence of HCN1-mediated feedback, the amplitude of rod signals remains at high levels for a prolonged period of time, leading to saturation of the retinal pathways and to the observed cone signal loss. To investigate the validity of this concept, we designed further experiments to assess the following derived hypotheses. Our first hypothesis was that, under conditions that lead to the loss of cone system signals, HCN1-deficient mice would show a sustained step response to rod stimulation, whereas control mice, owing to the internal photoreceptor feedback via HCN1 channels, would not. Second, we hypothesised that if rod function was selectively eliminated in HCN1 −/− mutants, the cone system would regain normal functionality. Finally, we hypothesised that, if the connections at which rods feed into the cone system were cut by genetic ablation of connexins or blocked pharmacologically, rod and cone systems would operate independently and cone function would be restored. First, we addressed the issue of prolonged rod responses, as this is the basis of our considerations. HCN1 −/− mice show persistent rod responses To investigate whether the lack of HCN1 leads to sustained and easily saturated rod ERG responses, we needed to compare the steady-state signal level during flicker to the baseline before onset of stimulation. In conventional ERG recording protocols, flicker responses are continuously averaged over time to improve signal-to-noise ratio, at the cost of losing baseline information. To retain this information, we recorded single traces of flicker ERG with a defined onset, and averaged those traces ( Fig. 5 ). To assure that we recorded rod system signals only, we used a sufficiently weak stimulus. 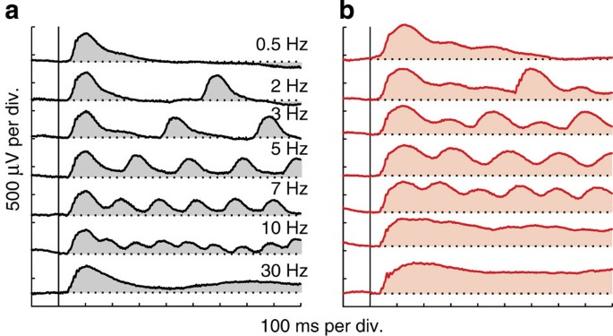Figure 5: Rod responses persist unphysiologically in HCN1−/−mice. Scotopic direct-current ERGs of a WT (a) and a HCN1−/−mouse (b). The vertical lines indicate the onset of flicker (that is, the time of the first flash of the sequence), and the horizontal dotted lines indicate the signal baseline. The prolongation of the waveform in the absence of HCN1 (b) led to a reduced flicker fusion frequency, together with an increasing failure of the rod ERG to reach baseline between flashes, culminating in a step-like response at higher flicker frequencies (approximately∼≥10 Hz). Figure 5: Rod responses persist unphysiologically in HCN1 −/− mice. Scotopic direct-current ERGs of a WT ( a ) and a HCN1 −/− mouse ( b ). The vertical lines indicate the onset of flicker (that is, the time of the first flash of the sequence), and the horizontal dotted lines indicate the signal baseline. The prolongation of the waveform in the absence of HCN1 ( b ) led to a reduced flicker fusion frequency, together with an increasing failure of the rod ERG to reach baseline between flashes, culminating in a step-like response at higher flicker frequencies (approximately ∼ ≥10 Hz). Full size image The resulting traces in Figure 5 support our view of rod signalling. In HCN1 −/− animals, the responses were considerably prolonged and saturation was reached at a much lower frequency. In particular, not only the flicker fusion frequency was higher in WT animals than in HCN1-deficient ones, but also the signal rapidly returned to lower levels, whereas the HCN1 −/− traces at stimulus frequencies above 10 Hz practically resembled a step response, corroborating our first hypothesis. A comparable step response was also present at the level of GCs (for example, Fig. 3c ). We therefore conclude that a sustained rod output signal in HCN1 −/− indeed leads to premature ON-bipolar saturation, and that HCN1 channel activity in WT animals precludes such saturation by modulating rod output, thereby increasing the remaining dynamic range of the system. Removal of rod responses restores cone signalling in HCN1 −/− We next assessed whether removal of rod output is sufficient to restore regular cone signals (second hypothesis). To ablate rod responses, we cross-bred HCN1 −/− mice with rhodopsin knockout animals [19] . The lack of rhodopsin precludes formation of rod outer segments, leading to the absence of rod signals. In contrast, the cone system functions normally until animals are about 5–6 weeks old and the secondary cone degeneration triggered by the loss of rods is manifested [20] . In ERG recordings of rho −/− mice ( Fig. 6a ), the lack of rod contributions is most apparent in the initial part of the frequency series because of the lack of a large a-wave and a reduction in b-wave [16] . 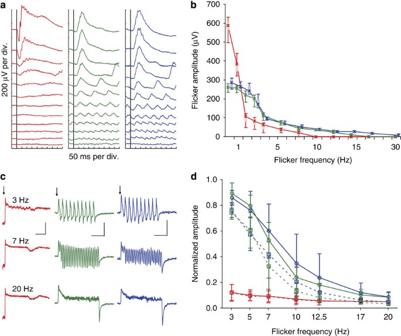Figure 6: Elimination of rod activity restores cone signalling. (a) Flicker ERG frequency series of a HCN1−/−(red), HCN1−/−rho−/−(green), and a rho−/−(blue) mouse. In the absence of rod system responses due the lack of rhodopsin, cone system function in HCN1 mutants is restored. Flicker frequencies from top to bottom were 0.5, 1, 2, 3, 5, 7, 10, 12, 15, 18, 20 and 30 Hz. (b) Box-and-whisker plot of flicker response amplitudes as in (a). Boxes indicate the 25 and 75% quantile range, whiskers indicate the 5 and 95% quantiles, and the asterisks indicate the median of the data (each groupn=4). (c) OFF-GC recordings from HCN1−/−(red), HCN1−/−rho−/−(green), and a rho−/−(blue) mice. Restoration of cone activity in current responses from OFF-GCs to mesopic flicker stimuli in the HCN1−/−rho−/−retina, comparable to that in single rho−/−retina. Flash duration: 20 ms. Flash intensity: 760 rhodopsin isomerizations per rod and flash (Rh* per rod*flash). Stimulus duration: 3 s (3 Hz), 3.5 s (7 and 20 Hz). Scale bars: horizontal 1s; vertical HCN1−/−0.2 nA, HCN1−/−rho−/−0.6 nA, rho−/−0.5 nA. (d) Resolution of flicker stimuli of GCs in the rho−/−(blue) and HCN1−/−rho−/−(green) retina, compared with HCN1−/−alone (red). ON-GCs (circles, solid lines) and OFF-GCs (squares, broken lines) were analysed separately (blue circles,n=5; green circles,n=5; blue squares,n=5; green squares,n=5). The normalized response amplitude is plotted against the stimulation frequency. Error bars indicate±s.d. around the mean. Normalized response amplitudes of both ON- and OFF-GCs did not differ between rho−/−and HCN1−/−rho−/−retina. Figure 6: Elimination of rod activity restores cone signalling. ( a ) Flicker ERG frequency series of a HCN1 −/− (red), HCN1 −/− rho −/− (green), and a rho −/− (blue) mouse. In the absence of rod system responses due the lack of rhodopsin, cone system function in HCN1 mutants is restored. Flicker frequencies from top to bottom were 0.5, 1, 2, 3, 5, 7, 10, 12, 15, 18, 20 and 30 Hz. ( b ) Box-and-whisker plot of flicker response amplitudes as in ( a ). Boxes indicate the 25 and 75% quantile range, whiskers indicate the 5 and 95% quantiles, and the asterisks indicate the median of the data (each group n =4). ( c ) OFF-GC recordings from HCN1 −/− (red), HCN1 −/− rho −/− (green), and a rho −/− (blue) mice. Restoration of cone activity in current responses from OFF-GCs to mesopic flicker stimuli in the HCN1 −/− rho −/− retina, comparable to that in single rho −/− retina. Flash duration: 20 ms. Flash intensity: 760 rhodopsin isomerizations per rod and flash (Rh* per rod*flash). Stimulus duration: 3 s (3 Hz), 3.5 s (7 and 20 Hz). Scale bars: horizontal 1s; vertical HCN1 −/− 0.2 nA, HCN1 −/− rho −/− 0.6 nA, rho −/− 0.5 nA. ( d ) Resolution of flicker stimuli of GCs in the rho −/− (blue) and HCN1 −/− rho −/− (green) retina, compared with HCN1 −/− alone (red). ON-GCs (circles, solid lines) and OFF-GCs (squares, broken lines) were analysed separately (blue circles, n =5; green circles, n =5; blue squares, n =5; green squares, n =5). The normalized response amplitude is plotted against the stimulation frequency. Error bars indicate±s.d. around the mean. Normalized response amplitudes of both ON- and OFF-GCs did not differ between rho −/− and HCN1 −/− rho −/− retina. Full size image With respect to cone signalling, the recordings in the HCN1 −/− rho −/− mice were practically indistinguishable from those in single rho −/− mutants. Notably, cone responses were observed at all stimulus frequencies, indicating that regular cone signalling was restored despite the continuing lack of HCN1 ( Fig. 6a,b ). This result obtained in vivo using ERG was confirmed in vitro using patch–clamp recordings ( Fig. 6c,d ). In both ON- and OFF-GCs, flicker stimuli of 3 and 7 Hz were equally well resolved in HCN1 −/− rho −/− and rho −/− animals. With these experiments, we have proven that removal of rod output was sufficient to restore regular cone signalling in HCN1 −/− mice, confirming our second hypothesis. Finally, we studied whether removal of functional connections between the rod and the cone system in HCN1 −/− animals would result in independent activity of both systems without the observed interference, thereby restoring cone signalling (our final hypothesis). Uncoupling of rod and cone pathways restores cone ERGs Rod and cone signals converge at several sites in the retina ( Fig. 1a,b ). So far, the only known essential component providing the electrical connections between rods and cones, as well as between cones, is the gap junction protein Cx36. Removal of such gap junctions in Cx36 −/− animals allows to study rod and cone system signals in the absence of direct rod–cone interactions, which are the basis for the secondary rod pathway. To eliminate these connections between rods and cones, we cross-bred HCN1 −/− animals with Cx36 −/− animals [21] . 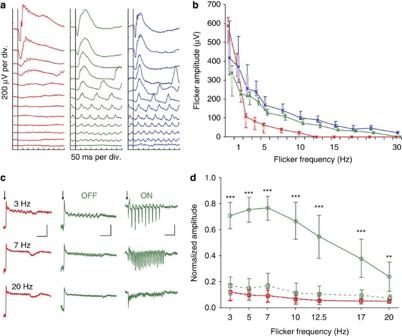Figure 7: Ablation of Cx36 gap-junction connections restores cone ON but not OFF signalling. (a) Scotopic flicker ERG frequency series of a HCN1−/−(red), a HCN1−/−Cx36−/−(green), and a Cx36−/−(blue) mouse. In the absence of Cx36 gap junctions, cone ERGs in HCN1 mutants are restored. Flicker frequencies from top to bottom were 0.5, 1, 2, 3, 5, 7, 10, 12, 15, 18, 20 and 30 Hz. (b) Box-and-whisker plot of flicker response amplitudes as in (a). Boxes indicate the 25 and 75% quantile range, whiskers indicate the 5 and 95% quantiles, and the asterisks indicate the median of the data (each groupn=4). (c) Current responses from OFF and ON-GCs in the HCN1−/−and HCN1−/−Cx36−/−retina to mesopic flicker stimuli. ON responses are restored in Cx36−/−or cx36-deficient deficient animals, whereas OFF responses are still suppressed. Flash duration: 20 ms. Flash intensity: 760 rhodopsin isomerizations per rod and flash (Rh* per rod*flash). Stimulus duration: 3 s (3 Hz), 3.5 s (7 and 20 Hz). Scale bars: horizontal 1s; vertical HCN1−/−, 0.2 nA, HCN1−/−Cx36−/−OFF 0.2 nA, HCN1−/−Cx36−/−ON 0.1 nA. (d) Resolution of flicker stimuli in the HCN1−/−retina (red) and HCN1−/−Cx36−/−retina (green) of ON-GCs (red circles,n=9; green circles,n=4; solid lines) and OFF-GCs (red squares,n=25; green squares,n=8; broken lines). The normalized response amplitudes are plotted against the stimulation frequency. Error bars indicate±s.d. around the mean. Note that normalized response amplitudes from ON-GCs in the HCN1−/−Cx36−/−retina differ significantly from those of ON-GCs in the HCN1−/−retina (***P<0.001; **P<0.01; 2-way ANOVA), while those of OFF-GCs do not. Figure 7a,b shows ERG data in the Cx36 −/− animals. Although the waveform shapes are slightly altered by the intervention with Cx36, both rod and cone system signal components can be clearly identified. In the HCN1 −/− Cx36 −/− double mutants, the rod-dominated part at low frequencies has a similar appearance to that of the single mutant Cx36 −/− mice. Compared with Cx36 −/− , light responses in the double knockout were prolonged, although not as pronounced as in HCN1 −/− . Strikingly, however, flicker frequency resolution in HCN1 −/− Cx36 −/− animals was indistinguishable from that of Cx36 −/− animals ( Fig. 7a,b ). Hence, regular cone signalling was restored in the ERG, but this time in the presence of rod signals (which however could not reach the cone pedicles via gap junctions, and, therefore, did not interfere with cone signals). Figure 7: Ablation of Cx36 gap-junction connections restores cone ON but not OFF signalling. ( a ) Scotopic flicker ERG frequency series of a HCN1 −/− (red), a HCN1 −/− Cx36 −/− (green), and a Cx36 −/− (blue) mouse. In the absence of Cx36 gap junctions, cone ERGs in HCN1 mutants are restored. Flicker frequencies from top to bottom were 0.5, 1, 2, 3, 5, 7, 10, 12, 15, 18, 20 and 30 Hz. ( b ) Box-and-whisker plot of flicker response amplitudes as in ( a ). Boxes indicate the 25 and 75% quantile range, whiskers indicate the 5 and 95% quantiles, and the asterisks indicate the median of the data (each group n =4). ( c ) Current responses from OFF and ON-GCs in the HCN1 −/− and HCN1 −/− Cx36 −/− retina to mesopic flicker stimuli. ON responses are restored in Cx36 −/− or cx36-deficient deficient animals, whereas OFF responses are still suppressed. Flash duration: 20 ms. Flash intensity: 760 rhodopsin isomerizations per rod and flash (Rh* per rod*flash). Stimulus duration: 3 s (3 Hz), 3.5 s (7 and 20 Hz). Scale bars: horizontal 1s; vertical HCN1 −/− , 0.2 nA, HCN1 −/− Cx36 −/− OFF 0.2 nA, HCN1 −/− Cx36 −/− ON 0.1 nA. ( d ) Resolution of flicker stimuli in the HCN1 −/− retina (red) and HCN1 −/− Cx36 −/− retina (green) of ON-GCs (red circles, n =9; green circles, n =4; solid lines) and OFF-GCs (red squares, n =25; green squares, n =8; broken lines). The normalized response amplitudes are plotted against the stimulation frequency. Error bars indicate±s.d. around the mean. Note that normalized response amplitudes from ON-GCs in the HCN1 −/− Cx36 −/− retina differ significantly from those of ON-GCs in the HCN1 −/− retina (*** P <0.001; ** P <0.01; 2-way ANOVA), while those of OFF-GCs do not. Full size image From these experiments we conclude that the connection between rods and cones is essential for the loss of cone signalling observed in the ERG of HCN1 −/− animals. These connections may also be important for the degree of prolongation of the light response. For example, cone circuits (that receive saturated rod responses in HCN1 −/− but not in the double knockout) might contribute to the prolongation of the light response. As cone signalling in the double knockout is observed at all frequencies, we further conclude that cone signals are reliably relayed to both ON- and OFF-bipolar cells. OFF-GC responses are still impaired in HCN1 −/− Cx36 −/− mice The ganglion cell recordings ( Fig. 7c,d ), however, revealed a striking difference in frequency resolution between the ON and the OFF channels. Whereas the ON channel showed normal frequency resolution, cone signals in the OFF channel were still impaired, indicating that the genetic ablation of Cx36 channels restored function at the level of ON-GCs but not OFF-GCs. We therefore reconsidered the signal flow involved in this situation. Transfer of rod signals to ON-GCs critically depends on Cx36 ( Fig. 8a ). Deletion of Cx36 abolishes signal transfer both via rod–cone coupling (secondary pathway) and via electrical synapses between AII and ON-cone bipolar cells (primary pathway). Hence, on knockout of Cx36, no rod signals can be conveyed to ON-GCs, leading to the restoration of normal cone flicker responses in the HCN1 −/− Cx36 −/− ( Fig. 7c,d ). 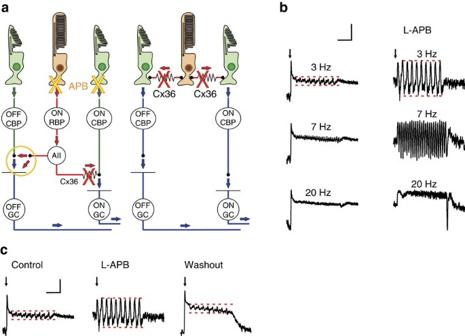Figure 8: L-APB treatment restores cone OFF signalling in the HCN1−/−Cx36−/−retina. (a) Rod signalling pathways in Cx36-deficient retina (cf.Fig. 1). Connections blocked by genetic ablation of Cx36 are marked with a red X. There is a complete separation between rod and cone ON pathways, but rod signals still have access to the cone OFF system via the primary rod pathway in the inner retina (marked with a yellow circle). Inactivation of the primary rod pathway by L-APB, specifically blocking the postsynaptic mGluR6 receptor in ON bipolar cells (sites marked with a yellow X), should thus restore cone OFF transmission. (b) Current responses to mesopic flicker stimulation from an OFF-GC in the HCN1−/−Cx36−/−retina under control conditions and during L-APB application. Under L-APB, the flicker frequency resolution in OFF-GCs is restored as predicted in (a). Flash duration: 20 ms. Flash intensity: 760 rhodopsin isomerizations per rod and flash (Rh*/rod*flash). Stimulus duration: 3 s (3 Hz), 3.5 s (7 and 20 Hz). Scale bar: horizontal 1 s, vertical 0.2 nA. (c) L-APB restored flicker resolution in OFF-GCs of HCN1−/−Cx36−/−mice in a reversible manner (that is, flicker resolution is lost on wash out of L-APB). Frequency 3 Hz; flash duration 20 ms; stimulus duration: 3 s; flash intensity: 760 rhodopsin isomerizations per rod and flash (Rh* per rod*flash). Scale bar: horizontal 1 s, vertical 0.2 nA. Figure 8: L-APB treatment restores cone OFF signalling in the HCN1 −/− Cx36 −/− retina. ( a ) Rod signalling pathways in Cx36-deficient retina (cf. Fig. 1 ). Connections blocked by genetic ablation of Cx36 are marked with a red X. There is a complete separation between rod and cone ON pathways, but rod signals still have access to the cone OFF system via the primary rod pathway in the inner retina (marked with a yellow circle). Inactivation of the primary rod pathway by L-APB, specifically blocking the postsynaptic mGluR6 receptor in ON bipolar cells (sites marked with a yellow X), should thus restore cone OFF transmission. ( b ) Current responses to mesopic flicker stimulation from an OFF-GC in the HCN1 −/− Cx36 −/− retina under control conditions and during L-APB application. Under L-APB, the flicker frequency resolution in OFF-GCs is restored as predicted in ( a ). Flash duration: 20 ms. Flash intensity: 760 rhodopsin isomerizations per rod and flash (Rh*/rod*flash). Stimulus duration: 3 s (3 Hz), 3.5 s (7 and 20 Hz). Scale bar: horizontal 1 s, vertical 0.2 nA. ( c ) L-APB restored flicker resolution in OFF-GCs of HCN1 −/− Cx36 −/− mice in a reversible manner (that is, flicker resolution is lost on wash out of L-APB). Frequency 3 Hz; flash duration 20 ms; stimulus duration: 3 s; flash intensity: 760 rhodopsin isomerizations per rod and flash (Rh* per rod*flash). Scale bar: horizontal 1 s, vertical 0.2 nA. Full size image In the OFF channel, only rod signals originating from the secondary pathway depend on Cx36. Rod signals in the primary rod pathway passing through rod bipolar cells and AII amacrine cells reach OFF-ganglion cells via glycinergic synapses. Therefore, removal of Cx36 leaves the primary pathway intact. We thus concluded that there is a need for a further dissection of pathways. Blocking the primary rod pathway restores cone OFF signalling As the rod–cone connection in the outer retina is not functional in the HCN1 −/− Cx36 −/− double mutant, we presumed that rod signals saturated the retinal network through the primary rod pathway ( Fig. 8a ). To confirm this hypothesis, we blocked the primary rod pathway in the HCN1 −/− Cx36 −/− retina using L-APB. L-APB acts as an agonist at the mGluR6 receptor expressed in rod bipolar cells and has been used in numerous studies to block the primary rod pathway (for example, see refs 22 , 23 ). A typical light response of an OFF-GC from the HCN1 −/− Cx36 −/− retina with strongly compromised flicker detection is shown in Figure 8b . On application of L-APB, flicker detection was fully restored in all OFF-GCs tested ( n =6). The effect was fully reversible after washout ( Fig. 8c ). From these results, we conclude that the effects created by loss of HCN1 on cone signalling and flicker resolution in OFF-GCs can be overcome when rod signalling in both primary and secondary rod pathways is eliminated. HCN1 channels were shown to be important for the shaping and shortening of photoreceptor voltage responses and for temporal filtering [24] , [25] . We found that deletion of HCN1 leads to prolonged rod responses in the ERG, together with a reduced flicker fusion frequency [13] . We concluded that this is due to the lack of HCN1 in rods, which is also supported by ex vivo tiger salamander data [26] and have developed a concept and a set of hypotheses to examine the nature of this phenomenon. We found that HCN1 channel feedback is of crucial importance under conditions when both rods and cones are active. The feedback helps to prevent saturation of the retinal network by rods during bright light stimulation. On ablation of HCN1, rod signals saturate the retinal network and obscure cone responses. Finally, rod signals interact with the cone system both in the inner retina via the primary rod pathway and in the outer retina via connexin 36-dependent rod–cone connections. In WT retina, HCN1 is expressed in rods, cones and several types of bipolar cells [13] , [27] . In principle, the deletion of HCN1 in any of these cell types could contribute to the loss of signalling under mesopic conditions investigated in this study. However, our results strongly indicate that the observed loss of cone signalling in HCN1 −/− is mostly due to the lack of HCN1 in rods. First, the loss of signalling was observed in all ON-GCs and all OFF-GCs, irrespective of the subtype. Hence, the cell type, whose HCN1 loss is responsible for the effect, must provide input into all ganglion cells and is, therefore, most probably a photoreceptor. In contrast, the loss of HCN1 in specific cone bipolar or amacrine cell types might only affect those ganglion cell types to which they are functionally connected. Second, in an intensity series, the loss of signalling was observed at illumination levels that saturate rods. Third, normal signalling is regained, if the rods are silenced (HCN1 −/− rho −/− ; Fig. 5 ). Finally, signalling is reconstituted, if the rods are functional but their pathways are blocked (L-APB in HCN1 −/− Cx36 −/− ; Fig. 8 ). From these experiments, we conclude that it is the deletion of HCN1 in rods that is responsible for the observed effect on retinal signalling. The deletion of HCN1 in other retinal cell types might result in effects that are either too subtle to be detected with our experimental design or are only apparent in subpopulations of ganglion cells. This needs to be addressed in further studies. The physiology of rods is governed by the interplay of several ion channel types. In the dark, CNG channel currents depolarize the rod, an effect that is counterbalanced by the potassium current I Kx (refs 28 , 29 ). Once the CNG channels are closed during bright light, I Kx draws the membrane potential towards hyperpolarized levels. Whereas, in WT photoreceptors, activation of HCN1 counterbalances strong hyperpolarizations, in the absence of HCN channel activity, the membrane potential may reach the potassium equilibrium potential E K (ref. 25 ). Moreover, high activity of the electrogenic Na + /K + -ATPase might hyperpolarize the membrane potential even further. It is still a matter of debate, whether inward-rectifying potassium channels exist in vertebrate photoreceptors. For example, in electrophysiological recordings of human rods [30] or monkey cones [31] , no inward-rectifying potassium currents were observed. However, they could be recorded in mouse rods [13] , [32] . Inward-rectifying potassium channels would prohibit hyperpolarization below E K . Therefore, E K may be the most negative membrane potential reached in mouse HCN1 −/− rods. The recovery from hyperpolarization would then depend on the speed of rise in cGMP in the outer segment followed by activation of CNG channels. Our study provides evidence that under mesopic conditions both primary and secondary rod pathways are active, and that rod and cone signals interact in both outer and inner retina. As the further knockout of Cx36 restored good flicker resolution in the ERG, we conclude that, on the level of bipolar cells, the secondary pathway was the main route for saturating signals. However, OFF-GCs in HCN1 −/− Cx36 −/− still showed saturated responses, which could be abolished by application of L-APB, and, therefore, were relayed via the primary pathway. While HCN1-mediated feedback rapidly modulates the photoreceptor membrane voltage, it does not drive rod output back to baseline, and, thus, does not entirely abolish saturation originating from the rod system. Under mesopic conditions, this saturation is evident in responses of WT GCs. Mesopic flicker stimulation induces a sustained current on top of which flash-induced current fluctuations and the OFF-response to the flicker stimulation ride ( Fig. 3c ). Our data suggest that this sustained current component originates from input by rod photoreceptors. First, it is not observed in rho −/− mice ( Fig. 6c ). Second, it is absent in ON-GCs of mice that lack Cx36 and, therefore, both primary and secondary rod pathway input to ON-GCs ( Fig. 7c ). Third, it can be abolished by L-APB that blocks the primary rod pathway in OFF-GCs of HCN1 −/− Cx36 −/− mice ( Fig. 8b ). In these three cases, the flicker response is better than in WT, irrespective of the presence or absence of HCN1 (compare rho −/− and HCN1 −/− rho −/− ; Fig. 6c ). In each neuronal network, saturation must be avoided. The retina has, therefore, developed very effective ways to adapt to stimulus changes over several orders of magnitude. Different adaptational mechanisms set in at different time points following stimulation. Examples for rather slow mechanisms are changes in the signal amplification of the phototransduction cascade and certain changes in the gain of synaptic transmission [33] , [34] . In contrast, HCN1 channel feedback provides a rapid adaptational mechanism that affects rod photoreceptor signals just past the leading edge. Activation of HCN1 channels feeds back onto photoreceptor membrane voltage, and hence synaptic output, within milliseconds. HCN1 is particularly well suited for this purpose as it shows the fastest activation of all HCN channels (for review see ref. 35 ). Ethical approval All procedures concerning animals adhered to the ARVO statement for the use of animals in ophthalmic and vision research and the law of animal experimentation issued by the German Government, and were performed with permission of local authorities (the Regierungspräsidium Tübingen and the Forschungszentrum Jülich). Mouse lines Wild-type, HCN1 −/− (refs 13 , 36 ), and Cx36 −/− (ref. 21 ) aged 4 weeks to 3 months, and rho −/− (refs 19 , 20 ), aged 4–5 weeks, were used in the experiments. We generated two types of double mutant mice by crossbreeding HCN1 −/− mice with rho −/− mice and Cx36 −/− mice, respectively, and subsequent breeding of each type of F1 heterozygotes. We identified double mutant mice in the F2 generation by PCR analysis of genomic DNA as described for the individual lines [19] , [21] , [36] . The resulting HCN1 −/− rho −/− and HCN1 −/− Cx36 −/− mice were examined at the age of 4–5 weeks. Electroretinography ERGs were performed using a Ganzfeld bowl, a direct current amplifier, and a PC-based control and recording unit (Multiliner Vision; VIASYS Healthcare) [17] . Mice were dark-adapted overnight and anaesthetized with ketamine (66.7 mg per kg body weight) and xylazine (11.7 mg per kg body weight). The pupils were dilated and responses to trains of flashes (flicker) for a fixed intensity (0.5 log cd s m −2 ; the ISCEV standard flash intensity [34] with varying frequency (0.5, 1, 2, 3, 5, 7, 10, 12, 15, 18, 20 and 30 Hz) were obtained under dark-adapted (scotopic) conditions using custom-made gold wire ring electrodes (Ø 0.25 mm). Flicker responses were averaged either 20 times (for 0.5, 1, 2, and 3 Hz) or 30 times (for 5 Hz and above). The flicker intensity series was done at a fixed frequency (6 Hz) with a range of intensities (−5.0 to 1.2 log cd s m −2 in steps of 0.2 logarithmic units). Band-pass filter cutoff frequencies were 0.3 and 300 Hz. The further ERG recording for the assessment of the absolute excitatory level of the retina induced by flicker of varying frequency was performed at a fixed, rod-specific stimulus intensity (−2 log cd s m −2 (ref. 16 )). Traces of 1 s length were obtained using direct-current signal amplification to avoid technical baseline alterations. Repetitive flashes were applied with a spacing in time mimicking the above flicker rates (0.5, 2, 3, 5, 7, 10 and 30 Hz) but having a defined onset. This way, the development of steady-state responses (towards the end of each trace) from the single flash response (at the beginning of stimulation) became accessible. Whole mount preparation for electrophysiology Light responses of GCs were recorded in vitro from retinal whole mount preparations. All steps were performed under infrared illumination using night vision equipment. Mice were dark-adapted overnight before they were deeply anaesthetized with isoflurane and decapitated. Eyes were rapidly enucleated and transferred to a dish containing oxygenized Ames medium. The cornea was cut along the ora serrata; the lens and vitreous were removed; and the retina was separated from the eyecup. Retinae were kept in Ames medium equilibrated with a mixture of 95% O 2 and 5% CO 2 (RT, pH 7.4) before electrophysiological recording. The tissue could be maintained for ≥4 h in oxygenated Ames medium. Electrophysiological recordings of GCs For the recording, the retina was mounted intact in a recording chamber with the photoreceptor side down. The tissue was continuously perfused with oxygenated Ames medium (32 °C, pH 7.4, 6 ml min −1 ). Cells were viewed on a video monitor coupled to a CCD camera mounted on a microscope (Zeiss) equipped with a water immersion objective (X40/0.80 W). The Nomarski optics of the microscope was modified for infrared illumination (≥850 nm). Patch clamp recordings of cells in the GC layer were performed in the whole-cell patch–clamp mode using an Axopatch-200A amplifier and pClamp8 software (Molecular Devices). GCs were identified by their electrophysiological properties, namely large sodium currents (>1 nA) and by their large somata. The intracellular solution consisted of (in mM) 126 KGlu, 10 NaCl, 4 KCl, 1 CaCl 2 , 1 MgCl 2 , 10 Na-HEPES, 10 EGTA, 1 Mg-ATP, 1 Na-GTP. Pipettes used for somatic recordings had resistances between 3 and 6 MΩ. Series resistances, which ranged from 10 to 30 MΩ, were left uncompensated. Drugs were diluted in Ames medium. Ames medium and all other chemicals were purchased from Sigma-Aldrich. To block rod responses via the primary rod pathway 50 μM L-APB (Tocris Cookson) was applied. Visual stimuli for electrophysiological recordings of GCs All visual stimuli were achromatic and presented on a 15-inch RGB colour monitor of a Windows XP computer. Stimuli were generated by a custom-made software kindly provided by Dr Thomas Euler (Centre for Integrative Neuroscience, University Tübingen, Germany). Stimuli were focused through the microscope condenser onto the photoreceptor cells and luminance was adjusted by neutral density filters ( I max ∼ 5×10 6 photons m −2 *s). Light spots that optimally stimulated the receptive field centre (100–200-μm diameter) were presented and light evoked currents were recorded from cells voltage–clamped to −60 mV. Flicker stimuli with different frequencies were used to determine the flicker resolution of individual GCs. Analysis Recordings were analysed using clampfit8 software (Molecular Devices). Every recording was repeated three times with 10-s breaks, and traces were averaged and filtered with a 50-Hz digital low-pass filter. To improve the signal to noise ratio, a data reduction (substitute average) was performed that reduced the sampling frequency from 10 kHz to 100 Hz. Frequency responses were analysed using homemade routines (Igor Pro, Wave-Matrics). Current amplitudes evoked by single flashes of the flicker stimulation were averaged (average modulation amplitude). The average modulation amplitude was divided by the maximal current amplitude (difference from the current peak at stimulus onset to peak at stimulus offset) to yield the normalized response amplitude. For the frequency-response function, normalized response amplitudes were plotted against the stimulus frequency. Numeric values are expressed as mean (±s.d.). Statistic analysis was performed with a 2-way ANOVA test or unpaired t -test. How to cite this article: Seeliger M.W. et al . Modulation of rod photoreceptor output by HCN1 channels is essential for regular mesopic cone vision. Nat. Commun. 2:532 doi: 10.1038/ncomms1540 (2011).